Dampened regulates the activating potency of Bicoid and the embryonic patterning outcome inDrosophila The Drosophila morphogen gradient of Bicoid (Bcd) initiates anterior–posterior (AP) patterning; however, it is poorly understood how its ability to activate a target gene may have an impact on this process. Here we report an F-box protein, Dampened (Dmpd) as a nuclear cofactor of Bcd that can enhance its activating potency. We establish a quantitative platform to specifically investigate two parameters of a Bcd target gene response, expression amplitude and boundary position. We show that embryos lacking Dmpd have a reduced amplitude of Bcd-activated hunchback ( hb ) expression at a critical time of development. This is because of a reduced Bcd-dependent transcribing probability. This defect is faithfully propagated further downstream of the AP-patterning network to alter the spatial characteristics of even-skipped ( eve ) stripes. Thus, unlike another Bcd-interacting F-box protein Fate-shifted (Fsd), which controls AP patterning through regulating the Bcd gradient profile, Dmpd achieves its patterning role through regulating the activating potency of Bcd. Embryonic patterning along the anterior–posterior (AP) axis of the Drosophila embryo is initiated by the action of the morphogenetic protein Bicoid (Bcd) [1] , [2] . Bcd is a transcriptional activator that stimulates the expression of AP-patterning genes [3] , [4] . One such gene is hunchback ( hb ), which, in response to the Bcd concentration gradient, has an expression domain in the anterior half of the embryo [5] , [6] . It is well documented that, based on morphological and molecular markers, altering the bcd gene dose maternally can shift the fatemap landscape in the embryo [7] , [8] . Experimental perturbations of the Bcd gradient properties such as the profile shape and precision can cause corresponding changes in the expression boundary of hb , further supporting a threshold-dependent action of Bcd in transcriptional activation during development [3] , [4] , [7] , [9] , [10] , [11] . Aside from its concentration-dependent action, there is another property of Bcd that is inherent to a transcriptional activator, namely, its ability (or potency) to activate target gene transcription. There have been studies investigating the activation domains of Bcd and the regulation of its activity [12] , [13] , [14] , [15] , [16] , [17] . However, it remains unknown—owing in part to a lack of adequate quantitative tools in the earlier studies—how the activating potency of Bcd may specifically have an impact on the AP-patterning network at a mechanistic level. F-box proteins play important regulatory roles in many molecular and cellular processes [18] , [19] , [20] , [21] , [22] . These proteins often exist as subunits of the SCF (Skp1-Cul1/Cdc53-F-box protein)-type ubiquitin E3 ligases, representing the specificity determinants of these protein complexes [22] , [23] , [24] . A well-documented function of F-box proteins is their ability to bind specifically to protein substrates and target them for ubiquitination and proteasome-mediated degradation. In a recent study, we reported the identification of a novel F-box protein, Fate-shifted (Fsd), that has a role in targeting Bcd for ubiquitination and degradation [10] . Embryos mutant for fsd have an altered (elongated) Bcd gradient profile and, as a result, a posterior shift in hb expression boundary and the entire fatemap. These results provide a fresh example illustrating the important roles of F-box proteins in regulating developmental fate specification. In addition to the regulation of substrate stability, F-box proteins have also emerged to have an ability to stimulate the activity of transcription factors [25] , [26] , [27] . For example, the F-box protein Skp2 can act as a co-activator for c-Myc-induced transcription in addition to regulating c-Myc stability [28] , [29] . Another F-box protein, β-TrCp1/Fbw1a, has been shown to enhance the ability of β-catenin to activate transcription through cooperating with the co-activator p300 in addition to targeting β-catenin for degradation [30] . We were interested in understanding whether the activating potency of Bcd might be subject to regulation by F-box proteins. A major motivation of our interest in this question lied at the promise that the Bcd gradient system should be suitable for dissecting the mechanistic details of transcriptional regulation in a native biological system with fine resolutions both temporally and spatially. Our analysis of Fsd indicated that this F-box protein does not regulate the activating potency of Bcd (see below for details), which is consistent with the fact that Fsd is predominantly localized to the cytoplasm [10] . Here we present studies of another novel F-box protein, encoded by dampened ( dmpd , CG11866), which is a nuclear cofactor of Bcd. We show that embryos from female mutants for dmpd have a decreased hb mRNA level at nuclear cycle (nc) 14, a defect that can be traced back to a reduction in hb -transcribing probability (hence, the gene name dampened ). The lowered amplitude (level) of hb expression can be propagated into the AP-patterning network to alter the spacing of even-skipped ( eve ) stripes that are sensitive to absolute concentrations of Hb. These results demonstrate that the activating potency of Bcd is subject to regulation for the embryo to achieve a normal AP-patterning outcome. The contrasting properties of Fsd and Dmpd also illustrate that two distinct properties of Bcd as a morphogen—its concentration gradient profile and its ability to activate transcription—are subjected to regulation by distinct F-box proteins. Nuclear F-box protein Dmpd regulates Bcd activity In our efforts to study the roles of F-box proteins in regulating Bcd functions, we identified Dmpd as a nuclear cofactor of Bcd. 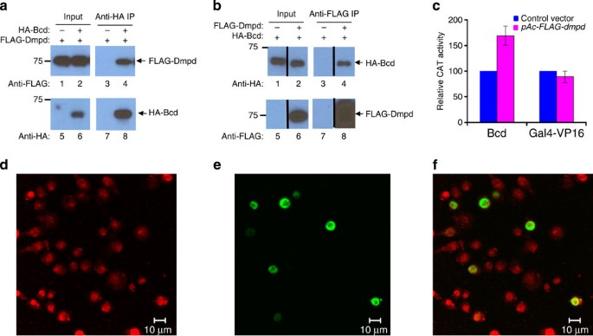Figure 1: Dmpd is a nuclear factor that stimulates Bcd-dependent reporter activity in cells. (a,b) FLAG-Dmpd interacts with HA-Bcd. co-IP experiments were performed to detect the interaction between FLAG-Dmpd and HA-Bcd. Here extracts from HEK293T cells expressing the indicated fusion proteins were subjected to co-IP by the indicated antibodies, followed by western blot detections by the indicated antibodies. Lanes 5 and 6 in these panels document the specificity of the antibodies used in our study. (c) Bcd activity is stimulated by Dmpd. Reporter assays were performed inDrosophilaS2 cells to evaluate the impact of Dmpd expression on CAT reporter activity. For each set of experiments, CAT activities were normalized to those obtained from cells without Dmpd expression (set as 100). Data shown are from three independent sets of experiments, with s.d. shown for Dmpd-expressing cells. (d–f) Nuclear localization of Dmpd. A plasmid expressing the HA-tagged Dmpd protein (HA-Dmpd) was transfected into S2 cells. Immunocytochemistry experiments were then performed to evaluate its subcellular localization through the use of the anti-HA antibody (e). To-pro-3 was used to counterstain the nucleus (d). Panelfis a merge of images shown in panelsd,e. Scale bar is 10 μm. Figure 1a,b shows the results of a co-immunoprecipitation (co-IP) assay, where we co-transfected the human embryonic kidney (HEK) 293T cells with plasmids expressing haemagglutinin (HA)-tagged Bcd (HA-Bcd) and FLAG-tagged Dmpd (FLAG-Dmpd). HEK293T cells are widely used as a host system to study F-box protein functions [10] , [31] . Here we used anti-HA antibody to pull down HA-Bcd in co-IP and anti-FLAG antibody to detect FLAG-Dmpd in western blots (see Fig. 1a,b , lanes 5 and 6, for control experiments documenting antibody specificity). Figure 1a shows the western blot results where FLAG-Dmpd was specifically co-precipitated by HA-Bcd (lane 4; see other lanes for controls). In a reciprocal setting, where anti-FLAG antibody was used to pull down FLAG-Dmpd in co-IP and anti-HA antibody was used to detect HA-Bcd in western blots, we obtained equivalent results ( Fig. 1b , lane 4, see other lanes for controls), further documenting an interaction between HA-Bcd and FLAG-Dmpd. Figure 1: Dmpd is a nuclear factor that stimulates Bcd-dependent reporter activity in cells. ( a , b ) FLAG-Dmpd interacts with HA-Bcd. co-IP experiments were performed to detect the interaction between FLAG-Dmpd and HA-Bcd. Here extracts from HEK293T cells expressing the indicated fusion proteins were subjected to co-IP by the indicated antibodies, followed by western blot detections by the indicated antibodies. Lanes 5 and 6 in these panels document the specificity of the antibodies used in our study. ( c ) Bcd activity is stimulated by Dmpd. Reporter assays were performed in Drosophila S2 cells to evaluate the impact of Dmpd expression on CAT reporter activity. For each set of experiments, CAT activities were normalized to those obtained from cells without Dmpd expression (set as 100). Data shown are from three independent sets of experiments, with s.d. shown for Dmpd-expressing cells. ( d – f ) Nuclear localization of Dmpd. A plasmid expressing the HA-tagged Dmpd protein (HA-Dmpd) was transfected into S2 cells. Immunocytochemistry experiments were then performed to evaluate its subcellular localization through the use of the anti-HA antibody ( e ). To-pro-3 was used to counterstain the nucleus ( d ). Panel f is a merge of images shown in panels d , e . Scale bar is 10 μm. Full size image Immunocytochemistry in Drosophila S2 cells reveals that Dmpd is almost exclusively localized to the nucleus ( Fig. 1d–f ), suggesting that it may play a role in regulating the function of Bcd as a transcriptional activator. To test this possibility, we used a reporter gene encoding chloramphenicol acetyltransferase ( CAT ) under the control of the ~250-bp Bcd-responsive native hb enhancer element [13] , [32] , [33] . Figure 1c shows that the CAT reporter activity was increased ~1.7-fold by the expression of Dmpd in cells. To determine whether the action of Dmpd on reporter activation might be through a general mechanism that is independent of Bcd, we performed reporter assays where the reporter expression is activated by an artificial transcription activator Gal4-VP16 (ref. 34 ). Our results ( Fig. 1c ) show that the reporter activity in this case was not increased by Dmpd expression in cells, excluding the possibility that Dmpd stimulates transcription through a general mechanism that is independent of Bcd. Evaluating hb expression boundary and amplitude To evaluate the impact of Dmpd on Bcd-activated transcription in a native developmental context, we first sought to establish a quantitative platform suitable for simultaneously but specifically evaluating the two parameters of a response to the Bcd input: the amplitude and boundary position of hb expression in the embryo. While previous studies in Drosophila embryos have focused extensively on the regulation of hb expression boundary [11] , [35] , [36] , [37] , [38] , [39] , [40] , relatively little attention has been paid to the regulation of the amplitude of Bcd target gene expression. We chose hb for evaluating the regulation of Bcd-activating potency because, unlike most AP-patterning genes that also respond to other inputs [41] , [42] , hb responds primarily to the Bcd input [9] , [43] , which should make it a sensitive target suitable for such evaluations. Gap genes such as hb are located at the top of the hierarchy of the regulatory cascade of the AP-patterning network to establish the earliest interpretations of the maternal inputs. For our experiments, we used quantitative fluorescence in situ hybridization (FISH) to detect mature hb mRNA in the cytoplasm of the blastoderm embryo. To maintain a linear relationship between the fluorescence signal intensity and hb mRNA level, we avoided any nonlinear signal amplification steps and ensured that all images were captured within a linear range. In addition, for any comparisons to be made, all the experimental and imaging steps were performed on a side-by-side basis. Under these conditions, the un-normalized, raw fluorescent intensities should allow us to compare directly the hb mRNA levels among different groups of embryos and, as detailed below, we used calibrating embryos to specifically validate this point. To process the captured images, we first extracted the FISH intensities at locations within the basal cytoplasmic layer along the dorsal side of an embryo. The extracted intensity data were then projected to the AP axis and expressed as a function of fractional embryo length (EL) x/L . For our study, we defined the hb expression boundary, x hb , as the AP position at which the detected FISH intensity is at half maximal. We quantify the amplitude of Bcd-activated hb expression through the use of hb plat , which denotes the averaged un-normalized, raw intensity at positions in the plateau region of the anterior hb expression domain of an embryo [44] . We used calibrating embryos to test and validate our quantitative platform outlined above. These embryos have one, two or four copies of the hb gene (referred to as 1 × , 2 × and 4 × hb embryos, respectively). Here side-by-side quantitative FISH experiments were performed in these embryos to detect and quantify mature hb mRNA. To ensure reliable comparison of hb expression properties, embryos were specifically selected to be at a time (~5–15 min into nc 14) when hb plat is known to have reached its stable, peak levels [44] . The only adjustment in our analysis was an embryo-specific background subtraction step that eliminated embryo-to-embryo differences in terms of background fluorescence. 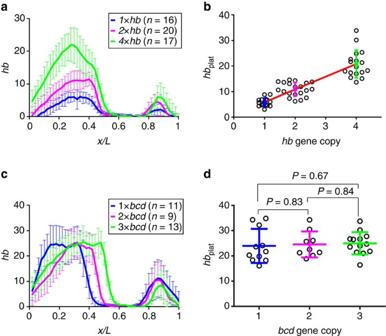Figure 2: Establishing a platform for quantifying the amplitude ofhbtranscription. (a) Shown are the mean profiles (with s.d. shown) of un-normalizedhbmRNA FISH intensities (in a.u.’s) from embryos that have one, two or four copies of thehbgene. The mean and s.d. ofxhbexpressed as fractional embryo length are: 0.435±0.013, 0.445±0.013 and 0.454±0.019 for 1 × , 2 × and 4 ×hbembryos, respectively (n=16, 20 and 17). These results show thatxhbremains largely insensitive to changes inhbcopy number in our experimental system; a relatively minor shift might be related to the limitations inherent to experimental detections35. (b) Shown arehbplatvalues (in a.u.’s) in individual embryos with different copies of thehbgene. The mean and s.d. are also shown in the figure (n=16, 20 and 17 for 1 × , 2 × and 4 ×hbembryos, respectively). The linear fit betweenhbplatandhbgene copy number is shown as a red line in the figure. (c) Shown are the mean profiles of un-normalizedhbmRNA FISH intensities in embryos from mothers with one, two or three copies ofbcd. The mean and s.d. ofxhbexpressed as fractional EL are: 0.373±0.013, 0.446±0.009 and 0.510±0.010 for 1 × , 2 × and 3 ×bcdembryos, respectively (n=11, 9 and 13). (d) Shown arehbplatvalues in individual embryos from mothers with different copies ofbcd. The mean and s.d. ofhbplatare: 23.93±6.75, 24.51±5.13 and 24.94±4.42 for 1 × , 2 × and 3 ×bcdembryos, respectively (n=11, 9 and 13).P-values (obtained from Student’st-tests and shown in the figure) reveal no significant differences. Figure 2a shows the mean hb intensity profiles from 1 × , 2 × and 4 × hb calibrating embryos (see Supplementary Fig. S1 . for individual intensity profiles). These profiles exhibit a classical and well-documented sigmoidal shape, each with a sharp boundary. Figure 2b shows that the mean hb plat values exhibit a linear relationship with the hb copy number ( hb plat =5.00 × c +0.86, where c is hb copy number; R squared for linear regression R 2 =0.75). These results show that hb plat detected under our experimental and analytical framework is a sensitive and reliable measure of the mature hb mRNA level and thus a valid parameter for quantifying the amplitude of a Bcd target gene response in the embryo. Figure 2: Establishing a platform for quantifying the amplitude of hb transcription. ( a ) Shown are the mean profiles (with s.d. shown) of un-normalized hb mRNA FISH intensities (in a.u.’s) from embryos that have one, two or four copies of the hb gene. The mean and s.d. of x hb expressed as fractional embryo length are: 0.435±0.013, 0.445±0.013 and 0.454±0.019 for 1 × , 2 × and 4 × hb embryos, respectively ( n =16, 20 and 17). These results show that x hb remains largely insensitive to changes in hb copy number in our experimental system; a relatively minor shift might be related to the limitations inherent to experimental detections [35] . ( b ) Shown are hb plat values (in a.u.’s) in individual embryos with different copies of the hb gene. The mean and s.d. are also shown in the figure ( n =16, 20 and 17 for 1 × , 2 × and 4 × hb embryos, respectively). The linear fit between hb plat and hb gene copy number is shown as a red line in the figure. ( c ) Shown are the mean profiles of un-normalized hb mRNA FISH intensities in embryos from mothers with one, two or three copies of bcd . The mean and s.d. of x hb expressed as fractional EL are: 0.373±0.013, 0.446±0.009 and 0.510±0.010 for 1 × , 2 × and 3 × bcd embryos, respectively ( n =11, 9 and 13). ( d ) Shown are hb plat values in individual embryos from mothers with different copies of bcd . The mean and s.d. of hb plat are: 23.93±6.75, 24.51±5.13 and 24.94±4.42 for 1 × , 2 × and 3 × bcd embryos, respectively ( n =11, 9 and 13). P -values (obtained from Student’s t -tests and shown in the figure) reveal no significant differences. Full size image Since hb expression is dependent on Bcd function, we sought to further document in an unambiguous manner whether hb plat is, or is not, sensitive to changes in bcd gene copies. Here our goal was to document specifically whether hb plat is sensitive to the hb boundary position or not. We performed quantitative FISH to detect hb mRNA in embryos from females that have one, two or three copies of the bcd gene (referred to as 1 × , 2 × and 3 × bcd embryos, respectively; see Supplementary Fig. S2 for individual intensity profiles). Figure 2c,d show our quantitative data. They confirm that x hb is a function of bcd gene copy number, exhibiting a progressive posterior shift as the bcd gene copy number increases. However, the mean hb plat values remain similar in 1 × , 2 × and 3 × bcd embryos ( Fig. 2d ). These results further document that hb plat quantifies exclusively how much hb mRNA is produced irrespective of where its expression boundary is located in the embryo. They provide further confirmation that hb plat is a valid and specific parameter for quantifying the amplitude of a Bcd target gene response. dmpd mutation reduces hb mRNA level in the embryo With the established quantitative platform outlined above, we proceeded to investigate the potential role of Dmpd in regulating the activating potency of Bcd during development. For this purpose, we generated a deletion allele dmpd 6-3 through P-element-mediated imprecise excision using a publicly available insertion line (Bloomington fly stock 17518). The resulting dmpd 6-3 allele has a 3,106-bp deletion covering almost the entire coding region of dmpd ( Fig. 3a ). It is homozygous viable at 25 °C, which made it possible for us to directly collect embryos from homozygous dmpd 6-3 females. Using our quantitative tools described above, we evaluated specifically the effect of the dmpd mutation on hb mRNA profiles in the embryo. Here we performed quantitative FISH in embryos from w 1118 or dmpd 6–3 mothers, referred to as wt and dmpd embryos, respectively. 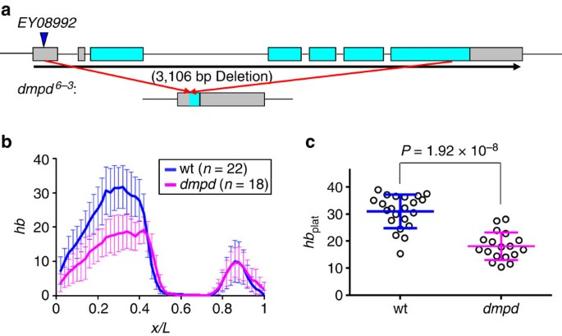Figure 3: ThehbmRNA level is reduced indmpdembryos. (a) A schematic diagram showing the deletion caused by thedmpd6-3allele. The boxes represent exons with the annotated open reading frame in cyan and the untranslated regions in grey. The blue arrow shows the P-element insertion site fordmpdEY08992. (b) Shown are the mean profiles of un-normalizedhbmRNA FISH intensities in wt anddmpdembryos (n=22 and 18, respectively). Note that the level of the Bcd-independent posteriorhbexpression domain remains unaffected indmpdembryos (P=0.93, Student’st-test); see text andclegend for further details). The mean and s.d. ofxhbexpressed as fractional embryo length are: 0.433±0.012 and 0.462±0.018 for wt anddmpdembryos, respectively (P=4.8 × 10−7, Student’st-test). (c) Shown arehbplatvalues in individual wt anddmpdembryos (n=22 and 18, respectively). Unlike the significant amplitude reduction for the Bcd-activated anteriorhbexpression domain shown in this figure, the amplitude of the Bcd-independent posteriorhbexpression domain,hbpost(defined as the average FISH intensities at the three peak positions of the posterior domain), is insensitive todmpdmutation. Figure 3b shows the mean profiles of hb mRNA FISH intensities (raw, background-subtracted) from wt and dmpd embryos (see Supplementary Fig. S3 for individual profiles), revealing a lower intensity level in dmpd embryos. Figure 3c shows that hb plat =30.98±6.18 (all values given in this report are mean±s.d. unless stated otherwise; n =22) and 18.10±5.10 ( n =18) in wt and dmpd embryos, respectively ( P =2.04 × 10 −8 ; all P -values given in this report are from Student’s t -tests unless stated otherwise), documenting a significant reduction in Bcd-activated hb expression amplitude in dmpd embryos. The observed defect of dmpd embryos in hb amplitude reduction is Bcd-dependent because the amplitude of the posterior hb expression domain, which is driven by a Bcd-independent enhancer [45] , was unaffected ( hb post =9.99±5.77 and 10.14±4.36 in wt and dmpd embryos, respectively; P =0.93; see Fig. 3c for hb post definition). In addition, the embryos chosen in our evaluation of hb mRNA levels are at early nc 14 since the hb expression stripe at parasegment 4 (PS4), which is dependent on gap gene cross-regulatory inputs [36] , [45] , has not yet gained any appreciable prominence ( Fig. 3b ). Together, these findings suggest that the activating potency of Bcd is subject to positive regulation by Dmpd during development. Figure 3: The hb mRNA level is reduced in dmpd embryos. ( a ) A schematic diagram showing the deletion caused by the dmpd 6-3 allele. The boxes represent exons with the annotated open reading frame in cyan and the untranslated regions in grey. The blue arrow shows the P-element insertion site for dmpd EY08992 . ( b ) Shown are the mean profiles of un-normalized hb mRNA FISH intensities in wt and dmpd embryos ( n =22 and 18, respectively). Note that the level of the Bcd-independent posterior hb expression domain remains unaffected in dmpd embryos ( P =0.93, Student’s t -test); see text and c legend for further details). The mean and s.d. of x hb expressed as fractional embryo length are: 0.433±0.012 and 0.462±0.018 for wt and dmpd embryos, respectively ( P =4.8 × 10 −7 , Student’s t -test). ( c ) Shown are hb plat values in individual wt and dmpd embryos ( n =22 and 18, respectively). Unlike the significant amplitude reduction for the Bcd-activated anterior hb expression domain shown in this figure, the amplitude of the Bcd-independent posterior hb expression domain, hb post (defined as the average FISH intensities at the three peak positions of the posterior domain), is insensitive to dmpd mutation. Full size image To evaluate the specificity of our dmpd deletion allele, we performed the following two sets of experiments. First, we compared hb plat between wt embryos and those from dmpd 6-3 / Df(2R)BSC303 females (referred to as dmpd/Df embryos). Df(2R)BSC303 is a small deficiency (~70 kb) that removes the entire dmpd -coding region. Our results ( Supplementary Fig. S4 ) show that, similar to dmpd embryos, dmpd/Df embryos also have a reduced hb plat from 25.05±5.47 ( n =10) in wt embryos to 17.93±4.03 ( n =12) in dmpd/Df embryos ( P =2.20 × 10 −3 ). Second, we backcrossed dmpd 6- 3 females with w 1118 males for six generations to establish a dmpd 6- 3 line in w 1118 background, referred to as dmpd 6-3w . We performed quantitative hb FISH in embryos from w 1118 or dmpd 6-3w females, further confirming a reduction in hb plat in dmpd 6-3w embryos ( Supplementary Fig. S5 ). In both sets of experiments, hb post was unaffected ( Supplementary Figs S4f,S5f ). Together, these results document that the observed hb plat reduction is a defect that is caused specifically by the dmpd mutation (as opposed to genetic background differences). They further support a role of Dmpd in stimulating specifically Bcd-dependent hb transcription in the embryo. dmpd mutation alters AP-patterning characteristics Hb regulates AP patterning by controlling the expression boundaries of downstream genes in a concentration-dependent manner [16] , [17] , [46] . Specifically, the spacing between the anterior boundaries of eve stripes 3 and 4 (referred to as ΔEL eve3-4 ) is known to be controlled by the absolute Hb concentrations in the embryo [47] , [48] . A reduction in the absolute Hb level (in hb /+ heterozygous embryos) has a well-documented consequence of enlarging ΔEL eve3-4 [47] , [48] . To determine whether the effect of Dmpd on hb transcription (that is, the reduced amplitude) can be propagated further downstream of the AP-patterning network, we performed quantitative FISH to detect eve expression patterns in wt and dmpd embryos for a direct comparison of ΔEL eve3-4 . 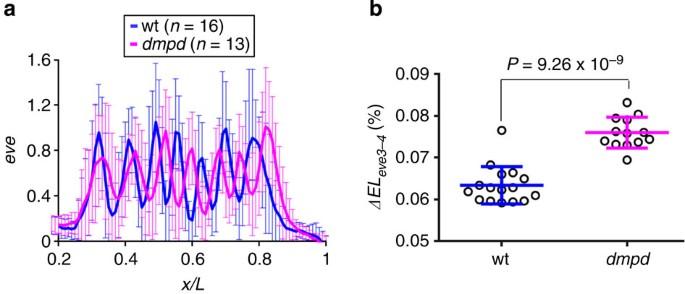Figure 4: The spacing betweenevestripes 3 and 4 is sensitive to thedmpdmutation. (a) Shown are the normalized mean intensity profiles ofevein wt anddmpdembryos (n=16 and 13, respectively). (b) Shown is the calculated distance betweenevestripes 3 and 4 in each individual wt anddmpdembryos (n=16 and 13, respectively). The distance values shown are expressed as percentage of embryo length. Also shown are the mean and s.d. for these two groups, along with theP-value obtained from Student’st-test. Figure 4a shows the mean intensity profiles of eve in wt and dmpd embryos (see Supplementary Fig. S6 for individual profiles). Figure 4b shows the measured ΔEL eve3-4 in these embryos, documenting a significantly larger ΔEL eve3-4 in dmpd embryos (7.60±0.37% EL, n =13) than in wt embryos (6.34±0.45% EL, n =16; P =9.26 × 10 −9 ). These results show that the impact of the reduced amplitude of hb expression caused by the dmpd mutation can be faithfully propagated downstream of the AP-patterning network, indicating a role of Dmpd in specifying a normal AP-patterning outcome. Figure 4: The spacing between eve stripes 3 and 4 is sensitive to the dmpd mutation. ( a ) Shown are the normalized mean intensity profiles of eve in wt and dmpd embryos ( n =16 and 13, respectively). ( b ) Shown is the calculated distance between eve stripes 3 and 4 in each individual wt and dmpd embryos ( n =16 and 13, respectively). The distance values shown are expressed as percentage of embryo length. Also shown are the mean and s.d. for these two groups, along with the P -value obtained from Student’s t -test. Full size image dmpd reduces hb -transcribing probability at nc 14 Our study described thus far shows that Dmpd can enhance the activating potency of Bcd and is required for a normal AP-patterning outcome. To investigate at a deeper mechanistic level how Bcd-activated hb transcription becomes compromised in dmpd embryos, we employed a technique that we developed recently for monitoring active hb transcription [44] . Here we used an intronic probe to detect the nascent hb transcripts near the Bcd-responsive P2 promoter (see Fig. 5a,b for images of a wt embryo at nc 14). Since the 283-bp hb intron is very close to the P2 promoter (145 bp downstream) and since RNA intron sequences are believed to be quickly removed upon being transcribed [49] , our technique permits a close monitoring of the transcriptional status of individual hb gene copies near the Bcd-responsive promoter. In our analysis, the fluorescence dots detected inside the nucleus (referred to as the intron dots) represent individual copies of hb undergoing active transcription in snapshots of the embryos. For each embryo, we first calculated the mean intron dot number per nucleus ( ρ ) at positions along the AP axis ( Fig. 5c ). This parameter quantifies the probability of hb gene copies undergoing active transcription (referred to as transcribing probability) at an AP position in a snapshot of the embryo. Specifically, ρ =2 indicates that all hb copies in the nuclei at the AP position under investigation are actively transcribing in the snapshot, thus denoting a transcribing probability of 100%. To specifically evaluate Bcd-activated hb transcription, we also calculated the average ρ for positions in the plateau region of the hb expression domain, ρ plat [44] . To minimize the effects of both PS4 and the variable anterior stripe [6] , [45] on the calculation of ρ plat , the plateau region was chosen to be a domain that spans 10% EL and has a posterior boundary that is ~10% EL anterior to the detected hb expression boundary of the embryo. The parameter ρ plat thus provides a quantification of the maximal Bcd-dependent transcribing probability of hb gene copies in a snapshot of the embryo. 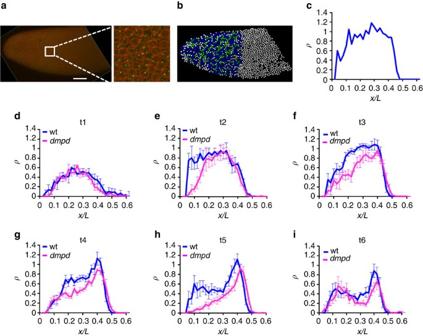Figure 5: The transcribing probability near Bcd-responsive promoter ofhbis decreased indmpdembryos. (a) Shown is an image ofhbintron staining from a cycle 14 embryo. Nuclear envelope is shown in red and intron dots in green. Scale bar, 50 μm. A magnified view of a section of the expression domain is shown on the right side of this panel. (b) Shown is a computer-processed image of panel (a). Here each of the identified nuclei is shown in a colour according to the number of intron dots detected inside. White, blue and green represent zero, one and two intron dots detected, respectively. (c) Shown is the plot ofρas a function ofx/Lbased on panelb. (d–i) Shown are the meanρprofiles from wt anddmpdembryos at time classes t1–t6. The mean and s.d. ofρplatfor t1–t6 time classes are: 0.50±0.07; 0.84±0.04; 1.03±0.08; 0.71±0.14; 0.52±0.10; 0.34±0.03 for wt embryos (n=3, 3, 7, 7, 5 and 4, respectively) and 0.51±0.11; 0.86±0.25; 0.79±0.21; 0.54±0.06; 0.38±0.12; 0.23±0.05 fordmpdembryos (n=3, 4, 5, 5, 5 and 4), respectively. TheP-values (from Student’st-tests) between wt anddmpdembryos for t1–t6 time classes are: 0.93; 0.92; 0.016; 0.028; 0.078; 0.0087, respectively. The meanρatx/L~0.15 (which is located outside of the plateau domain for calculatingρplat) appears higher indmpdembryos than in wt embryos at t6 (i); this is likely caused by an ‘outlier’dmpdembryo that has a very high level ofρat this location (seeSupplementary Fig. S8f). Figure 5: The transcribing probability near Bcd-responsive promoter of hb is decreased in dmpd embryos. ( a ) Shown is an image of hb intron staining from a cycle 14 embryo. Nuclear envelope is shown in red and intron dots in green. Scale bar, 50 μm. A magnified view of a section of the expression domain is shown on the right side of this panel. ( b ) Shown is a computer-processed image of panel ( a ). Here each of the identified nuclei is shown in a colour according to the number of intron dots detected inside. White, blue and green represent zero, one and two intron dots detected, respectively. ( c ) Shown is the plot of ρ as a function of x/L based on panel b . ( d – i ) Shown are the mean ρ profiles from wt and dmpd embryos at time classes t1–t6. The mean and s.d. of ρ plat for t1–t6 time classes are: 0.50±0.07; 0.84±0.04; 1.03±0.08; 0.71±0.14; 0.52±0.10; 0.34±0.03 for wt embryos ( n =3, 3, 7, 7, 5 and 4, respectively) and 0.51±0.11; 0.86±0.25; 0.79±0.21; 0.54±0.06; 0.38±0.12; 0.23±0.05 for dmpd embryos ( n =3, 4, 5, 5, 5 and 4), respectively. The P -values (from Student’s t -tests) between wt and dmpd embryos for t1–t6 time classes are: 0.93; 0.92; 0.016; 0.028; 0.078; 0.0087, respectively. The mean ρ at x / L ~0.15 (which is located outside of the plateau domain for calculating ρ plat ) appears higher in dmpd embryos than in wt embryos at t6 ( i ); this is likely caused by an ‘outlier’ dmpd embryo that has a very high level of ρ at this location (see Supplementary Fig. S8f ). Full size image To obtain an accurate comparison of hb- transcribing probability between wt and dmpd embryos, we grouped embryos into well-resolved temporal classes. These time classes have a temporal resolution of ~1 min with an uncertainty of ~0.6 to ~0.9 min (ref. 44 ). Figure 5d–i shows the mean ρ profiles in wt and dmpd embryos at time classes from t1 to t6 (see Supplementary Figs S7,S8 for individual profiles). These profiles show a reduced ρ level at time classes t3–t6, which represent embryos that are ~3 to ~6 min into nc 14 interphase (see Discussion for ρ properties at t1 and t2). For example, the peak transcribing probability is reached in wt embryos at t3 with a mean ρ plat of 1.03±0.08 ( n =7). By contrast, dmpd embryos at this time class have a significantly lower transcribing probability with a mean ρ plat of 0.79±0.21 ( n =5; P =1.6 × 10 −2 ; see Fig. 5 legend for P -values for other time classes). These results uncover an underpinning defect caused by the dmpd mutation, namely, a reduction in the transcribing probability of individual copies of the hb gene in the embryo. Importantly, the estimated contributions of active hb transcription at PS4 are insensitive to dmpd mutation in embryos that have developed a detectable PS4 stripe in the form of intron dots (see Supplementary Fig. S9 and legend). It is worth mentioning that, while the roles of cofactors in modulating the transcriptional outcome are well documented [50] , our finding that Dmpd regulates the transcribing probability of a native Bcd target gene in a native developmental system represents a significant advancement in our understanding of mechanisms of transcriptional regulation. dmpd does not affect Bcd gradient profile F-box proteins can enhance activator function through a variety of mechanisms [27] , [51] , [52] , [53] . They can be either proteolytic or non-proteolytic in nature as defined by their ability to regulate activator stability. To investigate whether Dmpd has a role in regulating Bcd degradation in addition to its co-activator function, we evaluated the Bcd gradient properties in dmpd embryos. Here we performed quantitative immunostaining to detect the Bcd protein in wt and dmpd embryos [10] , [11] . We extracted raw Bcd intensity without any adjustments, B , at different positions along the AP axis for individual embryos (see Supplementary Fig. S10 for the mean and individual profiles of Bcd intensities). According to a simple diffusion model, the length constant of an exponential Bcd gradient profile, λ , is a function of the diffusion constant D and degradation rate ω : λ 2 = D / ω (refs 38 , 54 ). In dmpd embryos, D is expected to be unchanged since Bcd itself is not altered, thus making it possible to use the estimated parameter λ to evaluate a potential impact of dmpd mutation on ω. 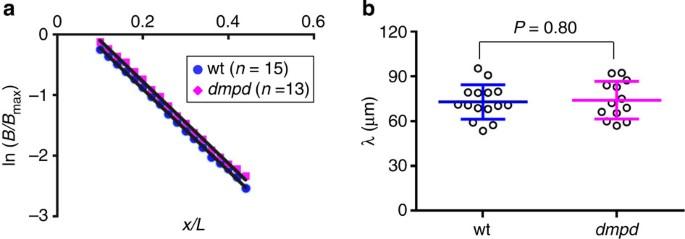Figure 6: Similar length constant of the Bcd gradient profiles in wt anddmpdembryos. (a) Shown are the mean Bcd gradient profiles from wt anddmpdembryos plotted asln(B/Bmax) against AP positionx/L. Here bothBandBmaxare background-adjusted intensities without any further adjustments. The solid lines represent linear fits (y=−6.78x+0.46,Rsquared for linear regression;R2=0.999 for wt embryos;y=−6.77x+0.58;Rsquared for linear regression,R2=0.998 fordmpdembryos). (b) Shown are calculatedλvalues of Bcd gradient profiles from individual wt anddmpdembryos (n=15 and 13, respectively). These values were obtained from fitting the individual Bcd intensity profiles to an exponential function. Shown are the mean and s.d. for these two groups, along with theP-value obtained from Student’st-test. Figure 6a shows ln( B/B max ) plots for the mean Bcd intensity profiles from wt and dmpd embryos (normalized to their respective mean maximal B value, B max ) as a function of x/L (see Fig. 6 legend for further details). Here the logarithmic conversion transforms an exponential profile to a linear profile, where λ is the negative reciprocal of the slope. Our results show that the two linear fits have a similar slope, suggesting a similar λ between wt and dmpd embryos. In a second analysis, we calculated λ values of Bcd gradient profiles from individual embryos (see Methods for details). Our results further confirmed the similarity of the length constant, λ =72.96±11.52 μm ( n =15) and 74.14±12.56 μm ( n =13) in wt and dmpd embryos, respectively ( P =0.80; Fig. 6b ). Together, these results suggest that, under the framework of a simple diffusion model, Dmpd does not have a significant role in regulating Bcd stability in embryos. They are supportive of a non-proteolytic role of Dmpd in enhancing the activating potency of Bcd. Figure 6: Similar length constant of the Bcd gradient profiles in wt and dmpd embryos. ( a ) Shown are the mean Bcd gradient profiles from wt and dmpd embryos plotted as ln(B/B max ) against AP position x/L . Here both B and B max are background-adjusted intensities without any further adjustments. The solid lines represent linear fits ( y =−6.78 x +0.46, R squared for linear regression; R 2 =0.999 for wt embryos; y =−6.77 x +0.58; R squared for linear regression, R 2 =0.998 for dmpd embryos). ( b ) Shown are calculated λ values of Bcd gradient profiles from individual wt and dmpd embryos ( n =15 and 13, respectively). These values were obtained from fitting the individual Bcd intensity profiles to an exponential function. Shown are the mean and s.d. for these two groups, along with the P -value obtained from Student’s t -test. Full size image Morphogen gradients such as those of Bcd are excellent experimental paradigms for dissecting the mechanistic operations of the regulatory networks that control patterning decisions. They provide a unique window to probing the regulatory impacts of F-box proteins both spatially and temporally at a fine resolution. Increasing evidence supports the notion that F-box proteins—there are up to 45 of them in Drosophila and 75 in humans [55] —belong to a critical class of regulatory proteins; however, few of them have been studied in native developmental contexts. In this work, we report the identification of a nuclear cofactor of Bcd, Dmpd, that can enhance the potency of Bcd as an activator. Dmpd thus joins an expanding list of F-box proteins that can act as transcriptional co-activators [28] , [29] , [30] ; it remains to be determined whether the co-activator role of Dmpd for Bcd in the embryo is dependent on a functional SCF complex and the E3 ligase activity. Our results show that embryos lacking Dmpd have a lower amplitude of Bcd-activated hb expression, a defect that can be passed further downstream of the network, causing an enlargement of ΔEL eve3-4 , the spacing between eve expression stripes that are sensitive to absolute concentrations of Hb. In embryos that lack another Bcd-interacting F-box protein Fsd, neither the hb expression amplitude nor ΔEL eve3-4 is affected ( Supplementary Fig. S11 ). This stems from the fact that, unlike Dmpd, Fsd regulates the Bcd gradient profile through a proteolytic pathway without a detectable co-activator function (Liu and Ma [10] and Supplementary Fig. S11 ). The contrasting functions of these two F-box proteins thus document that a normal AP-patterning outcome is subject to regulation by two distinct mechanisms. These mechanisms control two distinct properties of Bcd that are indispensable to its morphogen action: the formation of a concentration gradient and the activation of its target genes. A critical feature of morphogen gradients is their ability to induce downstream responses in a concentration-dependent manner. This particular feature has been subjected to extensive investigations, in part because of a significant interest in the question of what morphogen gradients do. It has been proposed recently that the concentration-dependent input–output relationship between Bcd and hb also contributes directly to the formation of AP patterns that are scaled with the length of the embryo [11] , [56] , [57] , [58] . By contrast, the regulation of the amplitude of a response to the morphogen input has been relatively underexplored. Its importance may be better appreciated from the perspective of regulatory networks that control the patterning outcome. In the case of hb as a direct target gene of Bcd, its encoded protein Hb acts as an input, in a concentration-dependent manner [47] , [48] , for genes (such as eve ) that are further downstream of the AP-patterning network. The regulation of the expression of these downstream genes allows the regulatory network to refine and evolve towards the desired final outcome of patterning. Since these downstream genes respond to absolute concentrations of Hb, the boundary position for hb expression in response to the Bcd gradient input has become no longer directly relevant to the decision-making processes of these genes. However, as shown by our study, another feature of the hb response to the Bcd gradient input, namely its expression amplitude, remains directly relevant to the continued operation of the AP-patterning network. Our analysis of the impact of the dmpd mutation on active hb transcription reveals important mechanistic insights into the regulation of the transcription process in a native developmental context. As documented recently [44] , Bcd-activated hb transcription becomes detectable immediately upon entering the nc 14 interphase; however, it is shut off within a few minutes. Our intron-staining results ( Fig. 5d,e ) show that, at time classes t1 and t2, the hb -transcribing probability at the plateau region is largely unaffected by the dmpd mutation (see Fig. 5 legend for ρ plat and P -values). They suggest that the onset of active hb transcription upon entering the nc 14 interphase is largely insensitive to dmpd mutation. The reduction in ρ plat at t3 and subsequent time classes is thus consistent with the possibility that dmpd embryos might have a hastened shutdown of active hb transcription at the nc 14 interphase. To test this possibility, we performed quantitative hb mRNA FISH in wt and dmpd embryos with an exclusive focus on nc 13. Embryos at this stage already have a significant accumulation of hb mRNA suitable for quantitative measurements that are necessary for effective comparisons between wt and dmpd embryos. In addition and importantly, active hb transcription is known to span the entire interphases prior to nc 14 (refs 44 , 59 ). Thus, if the defect of dmpd embryos is specific to hb shutdown at the nc 14 interphase, hb mRNA level should remain unchanged prior to this shutdown—that is, at nc 13. This prediction is supported by our results shown in Supplementary Fig. S12 . An implication of these findings is that altering the hb expression amplitude at, and only at, the last interphase (nc 14) prior to cellularization and gastrulation can still have an impact on the AP-patterning outcome, suggesting that this interphase represents a critical time period in making patterning decisions forward. An important feature of developmental systems is that their desired spatial properties must be attained within the allotted periods of time when an entire system is progressing along the irreversible temporal axis. This interconnection between the spatial and temporal aspects of the developmental systems poses significant constraints on their operation. In Drosophila , the early embryo undergoes rapid cycles of nuclear division [60] . This poses a constraint on the transcription process itself and the decoding of maternal gradient inputs, since mitosis is known to abort transcription [61] , [62] . It has been documented that active hb transcription can resume almost immediately upon entering the interphase in the blastoderm embryo [44] , [59] ; however, it remains unknown precisely how this can be achieved [61] . For developmental systems evolving rapidly along the temporal axis such as the early Drosophila embryo, patterning decisions may need to be made before true steady states could be achieved. In a recent study [63] , it was shown that how quickly a gene can resume efficient transcription upon entering the nc 14 interphase can affect the amount (the amplitude) of the gene products at a later time when such products are needed for action. Thus, it was shown that a slowed onset of snail transcription led to gastrulation defects [63] . In the case of dmpd mutation investigated in this report, while the onset of active hb transcription upon entering the nc 14 interphase is unaffected, a hastened shutdown reduces the amplitude of hb expression products, a defect that alters the spatial characteristics of the patterning outcome ( Fig. 4 ). Together, these two latest examples of dynamic regulation of transcription illustrate the importance of understanding the actual transcriptional decisions in a developmental system through the prism of time, an area of research that has only begun to be explored. Three recent studies have reported investigations of the dynamics of transcription in early embryos. Two of the studies [64] , [65] were based on a live-imaging technique using the MS2 coat protein system [66] , [67] . For evaluating the onset of transcription upon entering an interphase, the use of this system requires an adjustment by the delay between transcription initiation and detection of fluorescent signals at the reporter locus, as dictated by the time necessary for RNA polymerase to transcribe through the MS2 stem loop repeats and for the MS2 coat protein–green fluorescent protein to bind to these RNA repeats. With this and detection limit-imposed delay adjustments, both of the live-imaging studies are consistent with a quick onset of Bcd-dependent transcription initiation upon entering an interphase as documented in our current study and previous studies [44] , [59] . The live-imaging study of Lucas et al. [64] also supports a role of Bcd in directly lengthening the time period of active transcription during an interphase. At the nc 14 interphase, both the live-imaging study of Garcia et al. [65] and a third study of Little et al. [68] that was performed on fixed embryos support a shutdown of hb transcription that we initially reported [44] and further investigated in the current study. The results of Garcia et al. [65] , when adjusted by the method-dictated time delays, are also broadly consistent with our estimated kinetics of hb transcription onset and shutdown. Importantly, the observation [65] that a reporter gene driven by the ~250-bp Bcd-responsive hb enhancer element [13] , [32] , [42] is shut down at nc 14 in a manner that is broadly similar to the endogenous hb shutdown is consistent with our documented role of Dmpd and the activating potency of Bcd in influencing this shutdown process. Finally, we note that the dynamic properties of hb shutdown described by Little et al. [68] contradict with both our findings [44] and those of Garcia et al. [65] Unlike our experimental and analytical framework designed to evaluate specifically the dynamics of transcription initiation or elongation near the Bcd-dependent promoter [43] , [44] , [69] , the active hb loci detected by Little et al. [68] monitor the ‘aggregate’ transcription status along the entire hb gene length detected by the probes. This makes the fluorescent signal intensities at the active hb loci an insensitive quantity in studying the dynamics of hb shutdown at nc 14. In particular, the use of this quantity as transcription activity likely has contributed to the reported mismatch between ~30% reduction in ‘transcription activity’ and approximately threefold reduction in cytoplasmic hb mRNA counts from early to late embryos at nc 14. These results support a suggestion that, upon the sharp (in magnitude) and quick (in time) shutdown of hb transcription at early nc 14 as documented by our method [44] , the lingering signals at the ‘active’ hb loci [68] are largely unrelated to transcription initiation or elongation near the Bcd-dependent promoter. A contribution of our current work is the establishment of a quantitative platform for specifically (and simultaneously) analysing the amplitude and expression boundary of a target response to the Bcd gradient input. Under our current experimental framework, these two parameters are primarily subjected to regulation by two distinct mechanisms. Our results document that Dmpd has a role in enhancing the activating potency of Bcd as an activator and in regulating the AP-patterning outcome. Interestingly, we observe a detectable, although small, posterior shift in x hb in dmpd embryos (see Fig. 3 , Supplementary Figs S4,S5 , and their legends), suggesting that Dmpd may have regulatory roles beyond its primary role of regulating the amplitude of hb expression. This posterior shift in x hb cannot be simply explained by the Bcd gradient profile properties because a smaller B 0 (Bcd concentration at the anterior) in dmpd embryos, if biologically meaningful, would have predicted a small shift in x hb towards the anterior. This small shift is detectable in embryos not yet exhibiting a significant sign of PS4 expression ( Fig. 3 ), suggesting that it is related to Bcd-dependent hb transcription. It remains to be determined mechanistically whether Dmpd may have a meaningful role in regulating the affinity of Bcd for the hb enhancer during development. We anticipate that, as we develop more experimental tools and identify more regulatory players, we will be able to further improve our mechanistic knowledge about how the AP-patterning network operates in space and time at an even finer resolution and precision. Plasmids and lines of cells and flies Plasmids were constructed with standard DNA-cloning methods. To express proteins in Drosophila S2 cells and HEK293T cells, the corresponding cDNA sequences were cloned into the pAc5.1/V5-His C and pcDNA3 vectors, respectively. The following plasmids were from our previous studies [10] , [13] : FY441 expressing HA-Bcd from the pGEM3 vector, FY442 expressing HA-Bcd from the pAc5.1/V5-His C vector and ljb3087 expressing HA-Bcd from the pcDNA3 vector. The sequence encoding FLAG-Dmpd was PCR-amplified from a dmpd cDNA-containing clone (GM04147; the Drosophila Genomics Resource Center) with the following primers: 5′-GACTACAAGGACGACGATGACAAGATGGTGTCCACCCGCCAAATG-3′ (FLAG-Dmpd primer) and 5′-TGCTCTAGATTATTTACTGCGTTTGCCGGG-3′. The PCR product was digested with Xba I and ligated with the pGEM3 vector derived from FY441 that had been digested with Nco I, treated with the Klenow fragment of DNA polymerase I and digested subsequently with Xba I. The resulting intermediate plasmid, ljb4048, was then digested with Hin dIII and Xba I to yield a fragment (encoding FLAG-Dmpd) that was ligated with the pAC5.1/V5-His C and pcDNA3 vectors derived from Hin dIII and Xba I digestions of FY442 and ljb3087, respectively. The resulting plasmids ljb4049 and ljb4102 were used to express FLAG-Dmpd in Drosophila S2 and HEK293T cells, respectively. To obtain the plasmid (ljb4096) expressing HA-tagged Dmpd protein (HA-Dmpd) in Drosophila S2 cells, the same cloning strategy for ljb4049 was used, except for the use of an HA-tagged Dmpd primer (5′-GCTTACCCATACGATGTTCCAGATTACGCTATGGTGTCCACCCGCCAAATG-3′) in place of the FLAG-Dmpd primer. Drosophila S2 cells and HEK293T cells were grown in Schneider’s Drosophila medium (Invitrogen) at room temperature and Dulbecco’s modification of Eagle’s medium (Cellgro) at 37 °C, respectively. Both media contained 10% (v/v) fetal calf serum (Invitrogen) and 1 × antibiotic–antimycotic (Invitrogen). DNA transfection into both cells was performed using the FuGENE HD transfection reagent (Roche) according to the manufacturer’s instructions. Fly lines used for obtaining embryos with different hb gene copies were as follows: Df(3R)p13, red 1 , e 1 /TM3, Sb 1 (for 1 × hb embryos; Bloomington Drosophila Stock 1943); w 1118 (for 2 × hb embryos); KG-W25 (for 4 × hb embryos; a line kindly provided by Dr James W. Posakony [45] ). For the identification of 1 × hb embryos, we introduced a marked balancer chromosome ( TM3, hb-lacZ , which was derived from line no. 76 of the Bloomington Drosophila Stock Center) into the deficiency line to establish the Df(3R)p13, red 1 , e 1 /TM3, hb-lacZ, Sb 1 , Ser 1 flies. When these male flies were crossed to w 1118 virgin female flies, the desired 1 × hb embryos were identified by a lack of lacZ products. Female flies that contain different bcd gene copy numbers were as follows: Sp/CyO; bcd E1 /TM6B (for 1 × bcd embryos); w 1118 (for 2 × bcd embryos); Sp / CyO-bcd + ; Dr/TM6B (for 3 × bcd embryos; derived from a line kindly provided by Dr Gary Struhl [4] ). The fly line dmpd EY08992 (Bloomington Drosophila Stock 17518) was used in P-element-mediated imprecise excision to obtain the deletion allele dmpd 6-3 . The fly line w 1118 ; Df(2R)BSC303/Cyo (Bloomington Drosophila Stock 23686) is a deficiency line covering the entire dmpd -coding region. Immunocytochemistry and reporter assay Immunocytochemistry was performed [10] by first transfecting the HA-Dmpd-expressing plasmid into Drosophila S2 cells on a Lab-Tek II chamber slide. After fixing by 4% formaldehyde for 15 min at room temperature (RT), cells were permeabilized by 0.3% Triton X-100 and incubated with anti-HA antibody (1:100 dilution) at 4 °C overnight. After washing, Alexa Fluor488 goat anti-mouse IgG (1:400 dilution) was added to cells and incubated for 2 h at RT. TO-PRO-3 dye (1 μM) was added to stain DNA for 15 min at RT and, after washing, images were taken under confocal microscopy. Reporter assays were performed [70] by first transfecting Drosophila S2 cells with the hb-CAT reporter plasmid, the HA-Bcd-expressing plasmid, the copia-lacZ internal control plasmid, along with the FLAG-Dmpd-expressing plasmid (or pAc5.1/V5-His C as control). After 40 h post transfection, cells were harvested and lysed in 0.5% Triton X-100 by three freeze-thaw cycles. The lysates were added to a 150-μl mixture containing 0.2 M Tris-HCl, pH 7.5, 1.6 mM acetyl CoA (Sigma) and 0.25 μCi 14 C-Chloramphenicol (PerkinElmer), and incubated for 1 h at 37 °C. The amount of the lysate mixture used was adjusted by the transfection efficiency, which was evaluated by the β-galactosidase activity in the lysate. The products were extracted by adding 1 ml ethyl acetate, dried by a Speed Vac Concentrator and resuspended in 20 μl ethyl acetate. Ten microlitres of products were spotted in a plate for thin-layer chromatography (TLC) and allowed to migrate up the TLC plate with the chloroform: methanol (95:5) solvent. After being air-dried, the TLC plate was exposed to a storage phosphor screen (Molecular Dynamics) overnight. The screen was then scanned by the Storm 860 imaging scanner (Amersham) and intensities were quantified using the ImageQuant software. co-IP and western blots co-IP was performed [10] in HEK293T cells that had been co-transfected with plasmids expressing HA-Bcd and FLAG-Dmpd. The transfected cells were collected and lysed in the whole-cell extract buffer (400 mM KCl, 10 mM Na 2 HPO 4 , 1 mM EDTA, 1 mM dithiothreitol, 10% glycerol, 1 mM phenylmethylsulfonyl fluoride and 0.5% NP-40 with complete protease inhibitor cocktail). Appropriate antibodies and protein G Sepharose 4 fast flow beads were added to the extracts and mixtures were incubated overnight at 4 °C. After washing with the whole-cell extract buffer, the beads were boiled in 1 × SDS–PAGE loading buffer (50 mM Tris-HCl, pH 6.8, 100 mM dithiothreitol, 2% SDS, 10% glycerol and 0.1% bromophenol blue). Samples were loaded and separated using SDS–PAGE and transferred to Immun-Blot PVDF membrane (Bio-Rad). The membrane was then incubated with appropriate primary antibodies (1:1,000 dilution) followed by horseradish peroxidase-conjugated secondary antibodies (GE Healthcare, 1:2,000 dilution). Protein signals were visualized by the ECL plus western blotting detection reagents (GE Healthcare). HA-tagged and FLAG-tagged proteins were immunoprecipitated and detected by anti-HA (Covance) and anti-FLAG (Sigma) antibodies, respectively. Uncropped gel scans for western blot results are shown in Supplementary Fig. S13 . Imaging of stained embryos and data analysis All embryos used in this study were collected at 25 °C. Procedures of FISH to detect mRNA ( hb , lacZ and eve ), immunostaining to detect the Bcd protein and intron staining to detect hb nascent transcripts in the fixed embryos were as follows [10] , [11] , [44] . Fixed embryos were hydrated stepwise to PBST buffer and post-fixed by 10% formaldehyde for 20 min. After washing with PBST, embryos were transferred to the Hb-B buffer (50% formamide, 5 × SSC, 0.3% SDS and 0.1% Tween 20) stepwise and incubated with Hb-A buffer (50% formamide, 5 × SSC, 0.3% SDS, 0.1% Tween 20, 50 μg ml −1 heparin, 10 μg ml −1 yeast tRNA and 100 μg ml −1 denatured salmon sperm DNA) containing the appropriated Digoxigenin-11-UTP labelled RNA probes at 60 °C overnight. For anti-Bcd immunostaining, the overnight incubation at 60 °C was carried out in Hb-B buffer. The embryos were transferred back stepwise to PBST buffer at 60 °C and washed with PBST at RT for five times, followed by incubations first with 1.75 × blocking buffer (Roche) for a half hour and then with the primary antibodies (1:300 dilution of anti-Digoxigenin monoclonal antibody (Roche) for FISH and intron staining or 1:100 dilution of anti-Bcd antibodies (Santa Cruz Biotechnology) for immunotaining) at 4 °C overnight. After washing with PBST buffer, the embryos were incubated with 1.75 × blocking buffer for half an hour and then secondary fluorescence-conjugated secondary antibodies (1:400 dilution) for 1 h at RT. Individual embryos were assigned to a time class according to their mean nuclear height measured from the ‘lateral’ side of the midsagittal images [44] . Images for FISH and anti-Bcd immunotaining were captured with the Zeiss Imager Z1 ApoTome microscope on the midsagittal plane [10] , [11] , and those for intron staining were captured under confocal microscopy on the surface of the nuclear monolayer with serial z sections [44] . For FISH data analyses [10] , [44] , we first extracted raw intensities from the cytoplasmic layer using a circular window of 61 pixels to scan along the dorsal edge immediately outside of the nuclear layer (basally for hb ; apically for eve ). The scanning intervals were 2% EL for hb or 1% EL for eve along the AP axis of the embryo. The background used for subtraction in an individual embryo was the average intensity at a non-expression region (between the anterior domain and posterior stripe for hb ; the anterior 10% EL domain for eve ). To extract raw Bcd intensities from immunostained embryos, a circular window was used to scan the dorsal nuclear layer of the midsagittal images. To generate an intensity profile as a function of absolute distance from the anterior ( x ) or relative AP position ( x / L ), the scanning intervals were set as either ~12 μm or 2% EL. To calculate ρ from intron-staining data, all nuclei in an individual embryo were grouped into bins of the size of 2% EL along the AP axis. The average intron dot number per nucleus within each bin was calculated and defined as ρ . The measurement of EL required stitching two sets of images that were captured separately for the anterior and posterior parts of an embryo. The anterior ~60% EL domain for each embryo (where the intron-staining data were used in ρ calculations) was captured by a single set of images. To calculate the length constant ( λ ) of the Bcd gradient profile from an individual embryo, the equation of B = A × e – x /λ + C was used to fit the experimentally extracted data [10] . To avoid data from the non-exponential anterior region and the error-prone posterior region, fitting was performed within the x/L range of 0.2–0.9. Data fitting and other statistical analyses including Student’s t- tests (two-tailed) were performed using the Matlab software (MathWorks). How to cite this article: Liu, J. & Ma, J. Dampened regulates the activating potency of Bicoid and the embryonic patterning outcome in Drosophila . Nat. Commun. 4:2968 doi: 10.1038/ncomms3968 (2013).